Structure and function of lysosomal phospholipase A2 and lecithin:cholesterol acyltransferase Lysosomal phospholipase A2 (LPLA2) and lecithin:cholesterol acyltransferase (LCAT) belong to a structurally uncharacterized family of key lipid-metabolizing enzymes responsible for lung surfactant catabolism and for reverse cholesterol transport, respectively. Whereas LPLA2 is predicted to underlie the development of drug-induced phospholipidosis, somatic mutations in LCAT cause fish eye disease and familial LCAT deficiency. Here we describe several high-resolution crystal structures of human LPLA2 and a low-resolution structure of LCAT that confirms its close structural relationship to LPLA2. Insertions in the α/β hydrolase core of LPLA2 form domains that are responsible for membrane interaction and binding the acyl chains and head groups of phospholipid substrates. The LCAT structure suggests the molecular basis underlying human disease for most of the known LCAT missense mutations, and paves the way for rational development of new therapeutics to treat LCAT deficiency, atherosclerosis and acute coronary syndrome. Lysosomal phospholipase A2 (LPLA2, or group XV phospholipase A2) [1] and lecithin:cholesterol acyltransferase (LCAT) [2] are closely related secreted acyltransferases that transfer a fatty acid preferentially from the sn -2 position of glycerophospholipids to lipophilic alcohols or cholesterol, respectively ( Supplementary Fig. 1 ). LPLA2 is ubiquitously expressed but is most abundant in terminally differentiated alveolar macrophages [3] and is important for lung surfactant metabolism [4] and maturation of invariant natural killer T cells [5] . Inhibition of LPLA2 might be responsible for cellular toxicities caused by the administration of cationic amphiphilic drugs such as amiodarone [6] , and recent studies on LPLA2-knockout mice have linked LPLA2 to lupus erythematosus [1] and the innate immune response to infection by mycobacteria [7] . LCAT, 50% identical in amino-acid sequence to LPLA2, associates with high- and low-density lipoprotein (HDL and LDL) particles in plasma and catalyses an essential step in reverse cholesterol transport from peripheral tissues to the liver [8] . The acyltransferase activity of LCAT is responsible for the esterification of free cholesterol on discoidal pre-β-HDL particles, allowing their maturation into spherical α-HDL [9] . Genetic mutations of LCAT are responsible for somatic diseases such as familial LCAT deficiency (FLD), resulting from the complete loss of LCAT activity, and fish eye disease (FED) [10] , arising from the loss of LCAT activity towards substrates presented on HDL particles. Recombinant LCAT, together with artificial HDL particles, are being developed as potential therapeutics not only for the treatment of FLD [11] but also for atherosclerosis and acute coronary syndrome [12] . Despite over 60 years of research into the biochemistry of LCAT, the enzyme has remained structurally uncharacterized. Although predicted to contain a core α/β-hydrolase fold [13] , [14] , LPLA2 and LCAT have no close homologues of known structure. Herein are described multiple high-resolution crystal structures of LPLA2 along with a low-resolution structure of LCAT that confirms its close structural homology to LPLA2. These models provide a deeper understanding of the molecular mechanisms underlying substrate selectivity, catalysis and human disease in this important class of lipid-metabolizing enzymes. Atomic structure of LPLA2 The crystal structure of human LPLA2 ( Fig. 1a and Supplementary Fig. 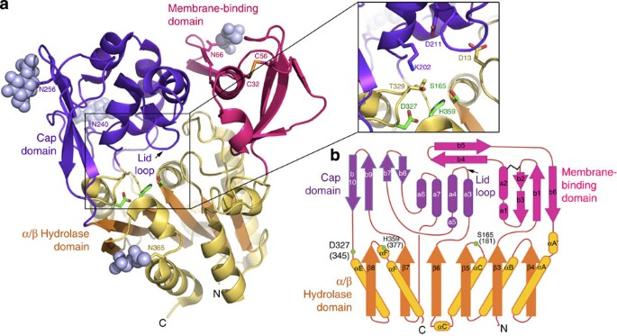Figure 1: Architecture of LPLA2. (a) The α/β hydrolase (gold with orange strands), membrane binding (magenta) and cap (purple) domains associate to form a large concave active site cleft. Catalytic triad residues are drawn with green carbons.N-acetylglucosamine sugars (light blue spheres) are observed at Asn66, Asn240, Asn256 and Asn365. The sole disulfide bond between Cys32 and 56 is drawn with yellow sulfur atoms. Inset displays a close up view of the catalytic triad region. (b) LPLA2 topology diagram. Because LPLA2 lacks the first two β strands of the canonical α/β hydrolase fold, the first strand of this domain is denoted as β3 (ref.19). Residues composing the LPLA2 catalytic triad are labelled and indicated with green spheres. To distinguish between α-helixes and β-strands composing the cap and membrane-binding domains from those in the α/β hydrolase domain, secondary elements of the latter domains are designated with Greek letters. LCAT has the same topology as LPLA2, and corresponding residue numbers are shown in parentheses. 2 ) was determined to 1.83 Å spacings using protein secreted from HEK293S GnTI − cells and deglycosylated with endoglycosidase F1 (endoF1) ( Table 1 and Supplementary Fig. 3a–d ). Experimental phases for the structure were obtained via single wavelength anomalous diffraction from crystals containing selenomethionine (SeMet)-labelled protein ( Supplementary Table 1 ). LPLA2 bears much closer structural similarity to Family I bacterial triacylglycerol lipases [15] (27 and 25% amino-acid sequence identity to the Bacillus subtilis and Pseudomonas aeruginosa lipases, respectively) than to other members of PLA2 superfamily [16] , such as cytosolic PLA2, calcium-independent PLA2 or platelet-activating factor acetylhydrolase. As in the bacterial lipases, it contains a six-stranded α/β hydrolase domain that lacks the first two strands of the canonical fold [17] and features a catalytic triad found at conserved topological positions: Ser 165 in a nucleophile elbow between β5 and αC, Asp 327 in a loop before αE, and His 359 in a loop following β8 ( Fig. 1b ). In addition, LPLA2 has a ‘cap’ domain formed by the β6–β7 and β7–αE loops of the α/β hydrolase domain. In the bacterial lipases, an analogous cap domain contributes to the ligand-binding site and features a flexible lid element that protects the active site from solvent and other potential ester substrates in the soluble form of the enzyme [18] , [19] . The LPLA2 cap domain is unrelated in fold, but contains two helices (α3 and α5) that are structurally analogous to two key helices found in bacterial lipase cap domains (α4 and α6), which contribute to the binding site for the scissile acyl chain of the lipid substrate ( Fig. 2 ). Figure 1: Architecture of LPLA2. ( a ) The α/β hydrolase (gold with orange strands), membrane binding (magenta) and cap (purple) domains associate to form a large concave active site cleft. Catalytic triad residues are drawn with green carbons. N -acetylglucosamine sugars (light blue spheres) are observed at Asn66, Asn240, Asn256 and Asn365. The sole disulfide bond between Cys32 and 56 is drawn with yellow sulfur atoms. Inset displays a close up view of the catalytic triad region. ( b ) LPLA2 topology diagram. Because LPLA2 lacks the first two β strands of the canonical α/β hydrolase fold, the first strand of this domain is denoted as β3 (ref. 19 ). Residues composing the LPLA2 catalytic triad are labelled and indicated with green spheres. To distinguish between α-helixes and β-strands composing the cap and membrane-binding domains from those in the α/β hydrolase domain, secondary elements of the latter domains are designated with Greek letters. LCAT has the same topology as LPLA2, and corresponding residue numbers are shown in parentheses. Full size image Table 1 Data collection and refinement statistics for crystal forms of LPLA2 expressed in HEK 293S GnTi − and treated with endoF1. 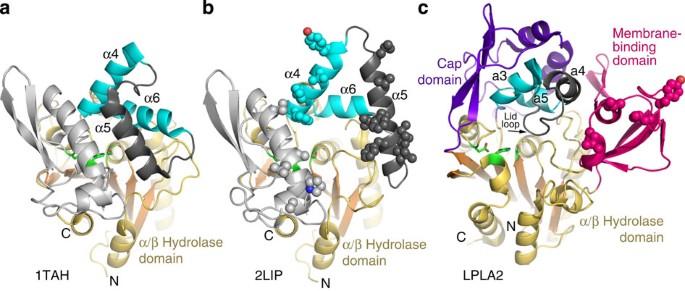Figure 2: Structural comparison of Family I triacylglycerol lipases with LPLA2. These enzymes all feature a similar α/β hydrolase core and cap domains that contain a topologically and structurally similar motif consisting of two helices (cyan) joined by a flexible loop (dark grey). In the bacterial lipase family, the α5 helix within this loop functions as an active site lid in the closed state and as a membrane-binding element in the open state. (a) Closed conformation of triacylglycerol lipase fromPseudomonas glumae(PDB entry 1TAH). (b) Open conformation ofPseudomonas cepacia lipase (PDB entry 2LIP). Potential membrane-binding residues are shown as spheres. (c) In comparison, LPLA2 seems to exhibit an open conformation, and the membrane-binding domain occupies a similar topological location with respect to the active site as the α5 helix in its open configuration inb. Hydrophobic residues predicted to be involved in membrane binding are shown as spheres. The lid loop and subsequent a4 helix of the cap domain (dark grey) is topologically equivalent to α5 ina,b. Full size table Figure 2: Structural comparison of Family I triacylglycerol lipases with LPLA2. These enzymes all feature a similar α/β hydrolase core and cap domains that contain a topologically and structurally similar motif consisting of two helices (cyan) joined by a flexible loop (dark grey). In the bacterial lipase family, the α5 helix within this loop functions as an active site lid in the closed state and as a membrane-binding element in the open state. ( a ) Closed conformation of triacylglycerol lipase from Pseudomonas glumae (PDB entry 1TAH). ( b ) Open conformation of Pseudomonas cepaci a lipase (PDB entry 2LIP). Potential membrane-binding residues are shown as spheres. ( c ) In comparison, LPLA2 seems to exhibit an open conformation, and the membrane-binding domain occupies a similar topological location with respect to the active site as the α5 helix in its open configuration in b . Hydrophobic residues predicted to be involved in membrane binding are shown as spheres. The lid loop and subsequent a4 helix of the cap domain (dark grey) is topologically equivalent to α5 in a , b . Full size image Unique to LPLA2, however, is a domain inserted in the loop between β3 and αA′ that contains the sole disulfide bond of the protein and a rare non-proline cis -peptide bond [20] between Trp43 and Leu44 that allows both of their hydrophobic side chains to project into the active site cleft. Relative to Family I bacterial lipases, the domain occupies a similar topological position as the lid element (α5) in its open configuration ( Fig. 2b,c ). The extended β4–β5 hairpin loop (residues 61–75) forms extensive interactions with the cap domain, burying 1,055 Å 2 of accessible surface area. Because this domain features a conserved hydrophobic surface that does not contribute to the active site ( Fig. 1a ) and mediates LPLA2 interactions with membranes (see below), it is henceforth referred to as the membrane-binding domain. The catalytic, cap and membrane-binding domains of LPLA2 assemble to form an extensive 1,240-Å 2 concave surface [21] containing the catalytic triad at the bottom, and each domain contributes surface exposed hydrophobic residues that should favor the binding of lipid reactants ( Supplementary Fig. 2b ). Compared with other lipases, which are known to have both active (open) and inactive (closed) conformations believed to be involved in interfacial activation [18] , [22] , access to the LPLA2 active site seems unimpeded except for a flexible 10 residue loop between the α3 and α4 helices of the cap domain, which is topologically equivalent to the larger lid elements found in Family I bacterial lipases ( Fig. 2 ). Because this element (henceforth referred to as the ‘lid loop’) is not highly conserved in sequence between LPLA2 and LCAT, it could play a role in determining their selectivity for N -acetylsphingosine (NAS) and cholesterol, respectively, as acyl acceptor substrates (see Discussion). Phospholipid substrate-binding site of LPLA2 Phospholipids and their analogues have not yet been successfully co-crystallized with either wild-type or catalytically inactive LPLA2-S165A. However, structures of LPLA2 bound to fluorophosphonate inhibitors are expected to mimic properties of the covalent intermediate of the reaction [23] ( Table 1 and Supplementary Fig. 4 ). The structures of LPLA2 bound to isopropyl dodec-11-enyl fluorophosphonate (IDFP; 2.3 Å spacings) and methyl arachidonyl fluorophosphonate (MAFP; 2.7 Å spacings) have a root mean squared deviation of 0.17 for 376 equivalent Cα atoms compared with ligand-free LPLA2, and thus the reaction with these compounds induces no major structural rearrangement despite increasing the melting point ( T m ) by 10–12 °C ( Supplementary Fig. 3e ). Omit map density reveals strong electron density for the MAFP and IDFP head groups, whose phosphonate groups are covalently bound to Ser165 and occupy the oxyanion hole formed by the backbone amides of Asp13 and Met166 ( Fig. 3a–c and Supplementary Fig. 4 ). The density, however, becomes progressively weaker after the C3 carbon of the alkyl chain. Heterogeneity in the position of the aliphatic tail of IDFP suggests that there are two distinct hydrophobic tracks (A and B) leading away from the catalytic triad ( Fig. 3a,b and Supplementary Fig. 5a ) that could correspond to the binding sites for the sn -1 and sn -2 acyl tails of the phospholipid substrate. Track A, which modelling indicates could readily accommodate at least 18 carbons, is curved and follows a hydrophobic band of residues on helices a3 and a5 in the cap domain, ending in a hydrophobic cleft formed by the side chains of Trp43, Trp57, Ile61 and Trp130. An unusual feature of this track is the presence of Asp13, which in bacterial lipases is conserved as either leucine or methionine. An alkyl chain occupying track A would therefore need to skirt around this residue to avoid unfavourable contacts, although in the low pH of the lysosome this residue should be at least partially protonated. 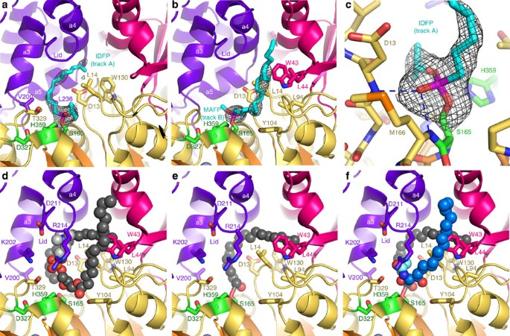Figure 3: Complexes with fluorophosphonate inhibitors help define the catalytic cycle of LPLA2. (a) IDFP (cyan sticks) occupying track A (seeSupplementary Fig. 5a). Wire cages ina–ccorrespond to 2.5σ|Fo|−|Fc| omit maps. (b) MAFP (cyan sticks) occupying track B. (c) Backbone amides of Asp13 and Met166 form the oxyanion hole of LPLA2 and coordinate the phosphonate group. (d) Model of POPC (spheres) bound in the active site such that itssn-2 chain occupies track A, andsn-1 chain track B. The head group (light grey spheres) is coordinated by Lys202, Asp211 and Thr329. (e) After dissociation of the lysophosphatidylcholine product, the acyl intermediate remains in track A, which would allow His359 to deprotonate an incoming alcohol nucleophile. (f) Model of NAS (blue spheres, cyan acetyl group) bound in track B. Figure 3: Complexes with fluorophosphonate inhibitors help define the catalytic cycle of LPLA2. ( a ) IDFP (cyan sticks) occupying track A (see Supplementary Fig. 5a ). Wire cages in a – c correspond to 2.5 σ | F o |−| F c | omit maps. ( b ) MAFP (cyan sticks) occupying track B. ( c ) Backbone amides of Asp13 and Met166 form the oxyanion hole of LPLA2 and coordinate the phosphonate group. ( d ) Model of POPC (spheres) bound in the active site such that its sn -2 chain occupies track A, and sn -1 chain track B. The head group (light grey spheres) is coordinated by Lys202, Asp211 and Thr329. ( e ) After dissociation of the lysophosphatidylcholine product, the acyl intermediate remains in track A, which would allow His359 to deprotonate an incoming alcohol nucleophile. ( f ) Model of NAS (blue spheres, cyan acetyl group) bound in track B. Full size image Track B is more solvent accessible and linear than track A, and begins adjacent to the oxyanion hole between the side chains of Leu14 (which contributes to both tracks) and Tyr104 in the catalytic domain, then extending along the surface of the membrane binding domain (including residues Trp43 and Leu44) in a channel formed between the lid loop of the cap domain, the αA′-αA loop of the catalytic domain, and the a1 helix of the membrane binding domain ( Fig. 3b and Supplementary Fig. 5a ). Although LPLA2 exhibits structural homology with bacterial lipases, their substrates are fundamentally different in that LPLA2 and LCAT hydrolyse glycerophospholipids, which contain polar, charged head groups, instead of triacylglycerol. Accordingly, there are modifications in conserved elements of the catalytic and cap domains of LPLA2 relative to the bacterial triacylglycerol lipases that seem to accommodate this difference. Lys202 in the a3 helix and Thr329 in the catalytic domain are invariant in LPLA2 and LCAT, but are conserved as hydrophobic residues in bacterial lipases. Modelling indicates that they could form specific hydrogen bonds with the phosphate in the phospholipid head group ( Fig. 3d ). The guanidinium of Arg214 in the lid loop is also in close proximity, although this residue is not conserved in LCAT. The K202A, N213Q/R214A and T329A mutations all retained full ability to hydrolyse the soluble substrate p -nitrophenylbutyrate (pNPB), indicating proper fold ( Fig. 4a ), but K202A and T329A were deficient in catalysing acyl transfer to NAS ( Fig. 4b ), consistent with Lys202 and Thr329, but not Arg214, being important for phospholipid binding. The side chain of Asp13 is also expected to be involved in substrate binding, perhaps by helping to dictate the course of acyl chains in track A. Accordingly, the D13A mutation decreased both soluble substrate pNPB hydrolysis and acyl transfer ( Fig. 4a, b ), suggesting that truncation of the side chain at this position disrupts the formation of favourable van der Waals contacts with the butyrate group of the substrate. 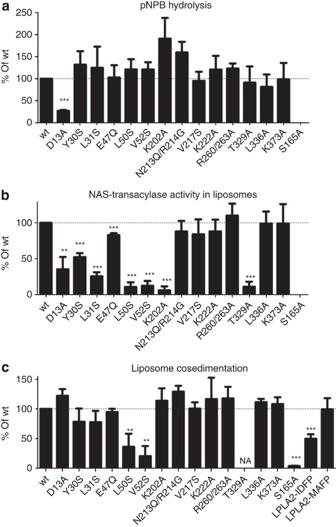Figure 4: LPLA2 enzymatic activity and liposome binding. (a) Hydrolysis of the soluble substrate pNPB at pH 7.5. Only D13A was significantly different from wild type (wt). (b) Transacylase assay using NAS-DOPC-sulfatide liposomes. (c) LPLA2 co-sedimentation with DOPC-sulfatide liposomes. LPLA2 was incubated with liposomes containing DOPC and sulfatide following ultracentrifugation. Amount of LPLA2 associated with membrane fraction was quantified and compared to wild-type (wt) LPLA2. Error bars represent the s.d. of three independent experiments. (**0.001<P<0.01, ***P<0.001. NA, not assayed due to poor protein expression; Student’st-test) Figure 4: LPLA2 enzymatic activity and liposome binding. ( a ) Hydrolysis of the soluble substrate pNPB at pH 7.5. Only D13A was significantly different from wild type (wt). ( b ) Transacylase assay using NAS-DOPC-sulfatide liposomes. ( c ) LPLA2 co-sedimentation with DOPC-sulfatide liposomes. LPLA2 was incubated with liposomes containing DOPC and sulfatide following ultracentrifugation. Amount of LPLA2 associated with membrane fraction was quantified and compared to wild-type (wt) LPLA2. Error bars represent the s.d. of three independent experiments. (**0.001< P <0.01, *** P <0.001. NA, not assayed due to poor protein expression; Student’s t -test) Full size image Conformational flexibility of LPLA2 Conformational flexibility is an important structural property of lipases, as interaction with a lipid bilayer is often thought to induce a conformational change that removes a lid covering the active site [24] . Among the eight unique crystal forms for LPLA2 reported here ( Table 1 and Supplementary Table 2 ), the most conformationally variable elements are the lid loop (residues 210–220), the αA′–αA loop (residues 96–102) and the a1 helix of the membrane-binding domain ( Fig. 5a ), consistent with their elevated temperature factors in the ligand-free structure ( Fig. 5b ). Interestingly, all three of these elements contribute residues to track B, suggesting that their structural plasticity allows for the binding of structurally distinct substrates, as is required by the catalytic cycle ( Supplementary Fig. 1 ). Sequence alignment of these regions in LPLA2 and LCAT reveals high conservation within each enzyme family, but less so between LPLA2 and LCAT ( Fig. 5c ), and thus these loops could also play a role in dictating acyl acceptor selectivity. However, despite many similarities to Family I bacterial lipases ( Fig. 2 ), none of the LPLA2 structures provide evidence for a large conformational change that would transition LPLA2 from a closed to an open state on membrane binding. 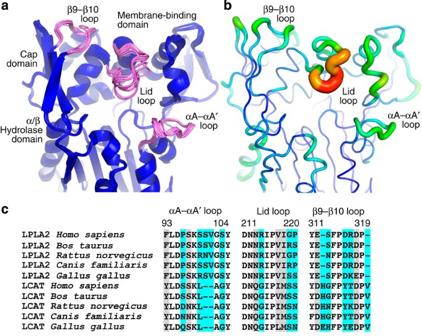Figure 5: Conformational and sequence variability in LPLA2. (a) Structural alignment of 16 unique LPLA2 chains from all of the unique LPLA2 crystal forms (Table 1andSupplementary Tables 1 and 2). Loops with highest root mean squared deviation scores (β9–β10 loop and lid loop of cap domain, and αA–αA′ of catalytic core) are shown in pink. (b) Temperature factor distribution is consistent with the conformational variability in panel A. Chain A of the ligand-free LPLA2 structure with B-factors indicated by colour (blue to red, 13 to 44 Å2) and by width of the Cα trace. (c) Sequence alignment of the most flexible LPLA2 loops with those of LCAT from the same species. Cyan and grey highlights indicate positions that are variable and highly conserved between LPLA2 and LCAT subfamilies, respectively. No highlight indicates invariance. Figure 5: Conformational and sequence variability in LPLA2. ( a ) Structural alignment of 16 unique LPLA2 chains from all of the unique LPLA2 crystal forms ( Table 1 and Supplementary Tables 1 and 2 ). Loops with highest root mean squared deviation scores (β9–β10 loop and lid loop of cap domain, and αA–αA′ of catalytic core) are shown in pink. ( b ) Temperature factor distribution is consistent with the conformational variability in panel A. Chain A of the ligand-free LPLA2 structure with B-factors indicated by colour (blue to red, 13 to 44 Å 2 ) and by width of the Cα trace. ( c ) Sequence alignment of the most flexible LPLA2 loops with those of LCAT from the same species. Cyan and grey highlights indicate positions that are variable and highly conserved between LPLA2 and LCAT subfamilies, respectively. No highlight indicates invariance. Full size image Membrane association of LPLA2 At lysosomal pH (~4.5), LPLA2 has an overall basic electrostatic surface that would complement the acidic inner leaflet of the lysosomal membrane ( Fig. 6a ). Examination of the structure also reveals a conserved, conspicuously solvent-exposed hydrophobic patch on the membrane-binding domain that includes Tyr30, Leu31, Leu50 and Val52 (conserved as Trp48, Met49, Leu68 and Leu70 in LCAT, respectively; Fig. 6a,b ). Mutation of these residues to serine had no significant effect on T m (data not shown) or on hydrolysis of the soluble substrate pNPB ( Fig. 4a ), indicating that these mutants were properly folded. However, all were impaired in acyl transfer ( Fig. 4b ) and liposome binding ( Fig. 4c ). Control surface mutations (for example, E47Q, V217S, K222A, R260/263A, L336A and K383A) had little or no significant effect in these assays. Taken together, these data are consistent with the existence of a specific membrane-binding site in the membrane binding domain. 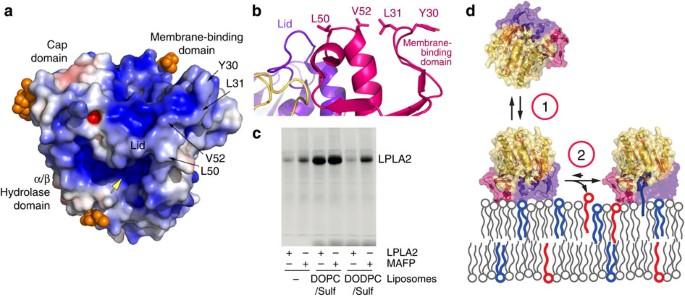Figure 6: LPLA2 membrane association. (a) Electrostatic surface potential (±5 kT e−1) of LPLA2 at pH 5. Glycosylation sites (orange spheres) would not sterically interfere with the interaction between the membrane binding domain and lipid bilayers. Yellow arrow indicates the entrance into the active site. (b) The membrane-binding surface of LPLA2. (c) LPLA2 requires either MAFP modification or substrate liposomes (DOPC-sulfatide) to stably associate with liposomes in pull down assays. Data shown are representative of four independent experiments. (d) Membrane association model. First, transient membrane binding is driven by complimentary electrostatic charge and the hydrophobic patch on the membrane binding domain. Second, formation of covalent acyl intermediate tethers LPLA2 at the membrane. Figure 6: LPLA2 membrane association. ( a ) Electrostatic surface potential (±5 kT e −1 ) of LPLA2 at pH 5. Glycosylation sites (orange spheres) would not sterically interfere with the interaction between the membrane binding domain and lipid bilayers. Yellow arrow indicates the entrance into the active site. ( b ) The membrane-binding surface of LPLA2. ( c ) LPLA2 requires either MAFP modification or substrate liposomes (DOPC-sulfatide) to stably associate with liposomes in pull down assays. Data shown are representative of four independent experiments. ( d ) Membrane association model. First, transient membrane binding is driven by complimentary electrostatic charge and the hydrophobic patch on the membrane binding domain. Second, formation of covalent acyl intermediate tethers LPLA2 at the membrane. Full size image Unexpectedly, the S165A mutation was completely deficient in membrane binding despite being indistinguishable from wild-type LPLA2 in T m ( Fig. 4c and data not shown) and in overall atomic structure ( Table 1 , data not shown). Because the LPLA2 active site is buried and relatively distant from the proposed membrane surface, we hypothesized that LPLA2 membrane association in liposome cosedimentation assays requires catalytic turnover. If so, then LPLA2 complexes with IDFP and MAFP, resembling the covalent intermediate step in LPLA2 catalysis, should stably associate with liposomes. The amount of the inhibitor-bound LPLA2 co-sedimenting with 1,2-dioleoyl- sn -glycero-3-phosphocholine (DOPC)-sulfatide liposomes was proportional to the length of the alkyl arm of the phosphonate inhibitor ( Supplementary Fig. 4 ) with LPLA2·IDFP retaining 50% and LPLA2·MAFP 100% of LPLA2 binding ( Fig. 4c ). Thus, the formation of an acyl intermediate seems to be a prerequisite for stable LPLA2 membrane association. If true, then liposomes lacking a substrate for LPLA2 should not support stable binding. In support of this theory, LPLA2 did not associate with 1,2- O -dioctadecenyl- sn -glycero-3-phosphocholine (DODPC)-sulfatide liposomes, which are not substrates for LPLA2, but LPLA2·MAFP could ( Fig. 6c ). Other catalytically deficient variants, however, still should be able to retain membrane interactions so long as an acyl intermediate can form. Indeed, the K202A mutation greatly decreases the rate of DOPC deacylation ( Supplementary Fig. 6 ) without impacting membrane binding ( Fig. 4c ). LCAT structure determination Compared with LPLA2, LCAT has amino (N)- and carboxyl (C)-terminal extensions that are not predicted to have significant secondary structure. However, the LCAT N-terminus (residues 2–5 of the mature protein) is known to be important for LCAT activity, possibly by mediating contacts with apolipoprotein A-I (ApoA-I) in HDL particles [25] . A glycosylated N-and C-terminally truncated variant of human LCAT (LCAT 21–397 ) exhibited similar activity on the soluble substrate pNPB and a similar T m as full-length LCAT ( Supplementary Fig. 7 ). This LCAT variant could also be crystallized, indicating that the N- and C-terminal extensions are not required for folding. An LPLA2-based homology model corresponding to the catalytic, membrane binding and cap domains of LCAT was then used to phase the 8.7 Å crystal structure of LCAT 21–397 by molecular replacement ( Fig. 7 and Table 2 ). The LCAT electron density maps revealed unbiased evidence for glycosylation at Asn84, Asn272 and Asn384, and all structural elements of the LCAT homology model fit well within the density envelope. Cys50 and 74, and Cys313 and 356, predicted to form disulfide bonds in LCAT, are in close enough proximity to each other to form covalent bonds ( Fig. 7c,d ). Residues of LCAT analogous to those in the hydrophobic membrane-binding patch in LPLA2 form a strong intermolecular crystal contact, wherein the Trp48 side chain of one chain binds deep into track B of a symmetry-related chain ( Fig. 7c ). The LCAT structure, albeit of low resolution, proves that the tertiary structure of LCAT is very similar to that of LPLA2 and has the same functional surfaces, permitting the extension of results from functional studies of LPLA2 to LCAT. 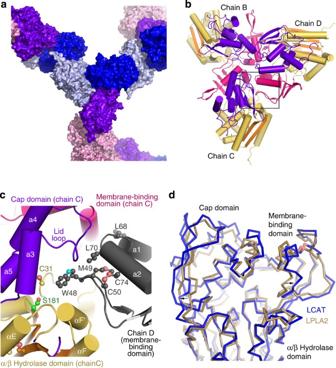Figure 7: Structure of human LCAT. (a) Surface representation showing lattice contacts in LCAT crystals, which contain 87% solvent (including sugar modifications estimated at 20 kDa (ref.55)). Each unique monomer in the asymmetric unit is coloured separately, and the four subunits form two homotrimers in the lattice, one non-crystallographic (chains B, C and D) and one crystallographic (chain A). (b) Non-crystallographic trimer formed by chains B, C and D. There is, however, no evidence for oligomerization of LCAT in solution as assessed by size exclusion chromatography (data not shown). Domains are coloured as for LPLA2 inFig. 1. (c) Crystal contacts exploit the predicted membrane binding patch of LCAT, which packs into track B of each three-fold symmetry related subunit. (d) Structural variance in the membrane binding and cap domains of LPLA2 (gold Cα trace) and LCAT (blue Cα trace). The catalytic domains of LCAT and LPLA2 were aligned. Structural elements of LCAT that bracket the active site (arrows) seem to expand outwards by up to 4 Å relative to LPLA2. Figure 7: Structure of human LCAT. ( a ) Surface representation showing lattice contacts in LCAT crystals, which contain 87% solvent (including sugar modifications estimated at 20 kDa (ref. 55 )). Each unique monomer in the asymmetric unit is coloured separately, and the four subunits form two homotrimers in the lattice, one non-crystallographic (chains B, C and D) and one crystallographic (chain A). ( b ) Non-crystallographic trimer formed by chains B, C and D. There is, however, no evidence for oligomerization of LCAT in solution as assessed by size exclusion chromatography (data not shown). Domains are coloured as for LPLA2 in Fig. 1 . ( c ) Crystal contacts exploit the predicted membrane binding patch of LCAT, which packs into track B of each three-fold symmetry related subunit. ( d ) Structural variance in the membrane binding and cap domains of LPLA2 (gold Cα trace) and LCAT (blue Cα trace). The catalytic domains of LCAT and LPLA2 were aligned. Structural elements of LCAT that bracket the active site (arrows) seem to expand outwards by up to 4 Å relative to LPLA2. Full size image Table 2 Data collection and refinement statistics for LCAT 21–397 . Full size table The structural and functional studies described above provide molecular explanations for the phospholipid and acyl acceptor selectivities exhibited by LPLA2 and LCAT. A typical preferred phosphatidylcholine (PC) substrate for LPLA2 contains a saturated acyl group in the sn -1 position (for example, palmitate), and an unsaturated, longer fatty acid (for example, oleic acid) in the sn -2 position ( Fig. 3d ) [26] . Consistent with this preference, the A and B tracks extending from the catalytic triad of LPLA2 adopt trajectories that match the physicochemical propensities of each of these acyl chains (that is, kinked versus linear, respectively). If the phosphate group of PC were constrained to interact with the side chains of Lys202 and Thr329, then the positively charged amine of the choline head group would be close enough to form favourable electrostatic interactions with the side chain of Asp211 in the lid loop, which is invariant in both LPLA2 and LCAT. Although LPLA2 has broad phospholipid head group selectivity [27] , LCAT is relatively specific for PC [28] and electrostatic interactions with the analogous residue (LCAT-Asp227) may be key for recognition of this lipid. LPLA2 favours lipophilic alcohol acyl acceptors, whereas the physiological acceptor of LCAT is cholesterol. Secondary alcohols such as cholesterol are not favoured as acyl acceptors in LPLA2, whereas aliphatic alcohols are less efficient acyl acceptors than sterols in LCAT [29] , [30] . Therefore, there must be distinct features in each of the LPLA2 and LCAT active sites that dictate this substrate preference. The most likely candidate based on sequence conservation and its topological position next to track B is the lid loop ( Fig. 5c ). The presence of a substantially larger and charged residue in LPLA2 (Arg214) relative to LCAT (Gly230) may discourage the binding of bulkier acyl acceptors such as secondary alcohols and sterols. Furthermore, the structural alignment of LPLA2 and LCAT based on their α/β hydrolase domains suggests that multiple structural elements around the active site are expanded in LCAT relative to LPLA2, as if to increase the volume of the active site cleft ( Fig. 7d ). Higher-resolution structures are required to validate this result. To test the role of the lid loop as a selectivity determinant, the LPLA2-N213Q/R214G mutant was assayed for cholesterol acyltransferase activity. Although this mutant had wild-type activity against soluble and lipid substrates ( Fig. 4a,b ), cholesterol ester formation could not observed under the acidic conditions required for LPLA2 catalysis on liposomes (data not shown). However, models of NAS and cholesterol bound to LPLA2 and LCAT, respectively, support the idea that the lid loop contributes to selectivity ( Supplementary Fig. 8 ). The modelling of each acceptor in the active site is constrained by the requirement for their nucleophilic hydroxyl groups to be close to the catalytic triad histidine as well as to LPLA2-Asp13/LCAT-Cys31, a position known to be important for cholesterol binding and activity regulation in LCAT [31] . Indeed, mutations at LCAT-Cys31, which serve to enhance LCAT activity, are being patented for the treatment of atherosclerosis and coronary heart disease [32] . The structural and functional studies reported herein also provide molecular insights into the LPLA2/LCAT catalytic cycle. We propose that LPLA2 first transiently interacts with the inner leaflet of the lysosomal membrane via favourable electrostatic [27] and hydrophobic interactions mediated by its membrane-binding domain ( Fig. 6d ). On membrane docking, a suitable phospholipid substrate enters the active site. The phospholipid acyl chain that binds in track A corresponds to the scissile chain, consistent with the structural homology of this acyl-binding site to the scissile site found in bacterial lipases and with the fact that the catalytic triad histidine is situated such that it can only protonate the lysophospholipid leaving group if it resides in track B ( Fig. 3d ). However, because LPLA2 has both phospholipase A2 and A1 activity, whether the sn -1 or sn -2 chain binds in track A also depends on its structural properties (that is, size and curvature). Indeed, LPLA2 prefers to transfer oleic (C18:1) and linoleic (C18:2) fatty acids [26] perhaps because their length and unsaturation enables them to pack more efficiently in track A. When POPC is modelled into the active site of LPLA2 with its oleic group in sn-2 position occupying the track A, the cis -9 double bond occupies the position opposite Asp13 and facilitates packing into the curved binding pocket. Asp13 is conserved as Cys31 in LCAT, a residue well known as being important for cholesterol binding and modulation of LCAT catalytic activity [31] , [32] , [33] . Interestingly, the pK a of cysteine is such that Cys31 will likewise be partially deprotonated in human plasma (pH 7.4). Acyl intermediate formation serves to retain the enzyme at the membrane until an appropriate lipophilic acyl acceptor enters the active site ( Fig. 6d ). After dissociation of the lysophospholipid product ( Fig. 3e ), the more accessible track B is left open for binding water (corresponding to lipase activity) or lipophilic alcohols (corresponding to acyl transferase activity; Fig. 3f ). A model of NAS docked into track B of the LPLA2 active site potentially explains the preference of the enzyme for lipophilic alcohols with a short side chain, such as C2 ceramide [29] , because this group would project towards the acyl-intermediate bound in track A ( Fig. 3f , Supplementary Fig. 8a ). Residues that coordinate the phosphate of the PC head group may also form specific hydrogen bonds with the N -acetyl group of NAS. After product release, LPLA2 most likely dissociates from the membrane until the next catalytic cycle, analogous to LCAT dissociation from HDL particles triggered by product release [34] . High-resolution structural characterization of the LPLA2/LCAT family provides a much deeper understanding of the molecular defects underlying 53 missense mutations in human LCAT that lead to FED and FLD ( www.lcat.it ). Supplementary Table 3 lists these mutations along with their clinical phenotype (FLD or FED, but note that assigning phenotype is often complicated by late onset of symptoms, compound heterozygosity or environmental factors) and relative levels of activity on HDL and LDL particles. Many FLD mutations result in structural defects that likely impact the folding, processing, and/or structural stability of LCAT ( Fig. 8a and Supplementary Fig. 9a ). These include defects in the core of the catalytic domain such as V28M, T106A, E110D, Y111N, R135Q/W, R140H/C, A141T, Y144C, Y156N, L209P, A211T, P307S, V309M, C313Y, L314F and L372R, or of the cap domain such as R244H/C and T274A/I (the latter of which is also likely a glycosylation defect). FLD-causing mutations are located in the interface between the β4–β5 loop of the membrane-binding domain and the cap domain (V90M, S91P and M293R/I), supporting the idea that this belt-like interdomain contact is critical for the overall fold of the enzyme. An inactivating R147W mutation is localized to the interface between the membrane-binding and catalytic domains, suggesting that the integrity of this contact is also important for function. 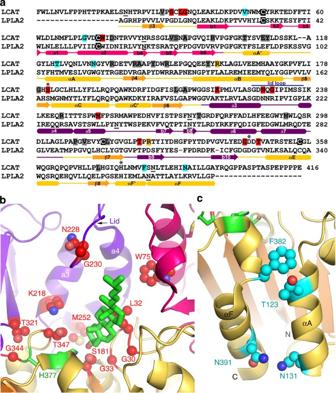Figure 8: FLD and FED somatic mutations of LCAT. (a) Sequence alignment of mature human LPLA2 and LCAT. Mutated positions predicted to have structural defects are highlighted grey, catalytic defects red, HDL-binding defects cyan and undetermined yellow. Cysteines involved in disulfide bonds are highlighted in black.N-linked glycosylation sites are underlined. Purple line indicates the lid loop of LPLA2. (b) Mutations affecting the LCAT active site (side chains shown as red spheres) cluster around the catalytic triad (green carbons) and predicted cholesterol (green stick model) binding site. (c) FED mutations (side chains shown as cyan spheres) tend to be found on the surface of the protein. The most prominent cluster is localized on the catalytic domain close to the N and C-termini of the enzyme. Figure 8: FLD and FED somatic mutations of LCAT. ( a ) Sequence alignment of mature human LPLA2 and LCAT. Mutated positions predicted to have structural defects are highlighted grey, catalytic defects red, HDL-binding defects cyan and undetermined yellow. Cysteines involved in disulfide bonds are highlighted in black. N -linked glycosylation sites are underlined. Purple line indicates the lid loop of LPLA2. ( b ) Mutations affecting the LCAT active site (side chains shown as red spheres) cluster around the catalytic triad (green carbons) and predicted cholesterol (green stick model) binding site. ( c ) FED mutations (side chains shown as cyan spheres) tend to be found on the surface of the protein. The most prominent cluster is localized on the catalytic domain close to the N and C-termini of the enzyme. Full size image Other inactivating mutations perturb the catalytic machinery ( Fig. 8b and Supplementary Fig. 9b ). The backbone amides of Cys31 and Leu182 form the oxyanion hole in LCAT, and mutation of residues in close proximity such as G30S, L32P and G33R consequently all produce FLD phenotype in human patients. The G179R, S181N and G183S mutations eliminate the activity by either removing the catalytic nucleophile or perturbing the nucleophile elbow that supports the active site serine, as previously predicted [35] . Another class of mutations supports the assigned roles of tracks A and B and of residues proposed to coordinate the phospholipid head group ( Fig. 8b and Supplementary Fig. 9b ). The G33R mutation, if it folds, would obstruct track B and block acyl acceptor binding. The W75R and M252K mutations would introduce positive charge into track A. T347M, which leads to almost complete loss of LCAT activity on HDL- and LDL-bound cholesterol when expressed in vitro [36] , is consistent with the catalytic defects exhibited by LPLA2-T329A. The LCAT K218N mutation, which results in full loss of activity [37] , is likewise consistent with catalytic defects exhibited by the LPLA2-K202A mutation ( Fig. 4a,b ). Mutations in the lid loop also generate the FLD phenotype [38] , [39] . N228K and G230R (which, interestingly, converts the latter position to its equivalent in LPLA2) greatly diminish the activity of LCAT, consistent with a role in substrate binding. Of particular interest are mutations of residues on or near the surface of LCAT that do not have a clear structural explanation for loss of activity and/or have an FED phenotype ( Fig. 8c and Supplementary Fig. 9c ). The V46E and G71R mutations are located in the membrane-binding domain, in close proximity to the proposed membrane-binding surface, and likely disrupt interactions with phospholipid bilayers. The T123I, N131D, R135Q/W, F382V and N391S mutations are located on a contiguous surface of the catalytic domain spanning helices αA′, αA and αF ( Fig. 8c ). This region is therefore also in close proximity to the N-terminal extension of LCAT, which is known to be important for activity on HDL [25] , and may represent a macromolecular interaction site for HDL particles, consistent with prior site-directed mutagenesis and antibody-binding experiments [40] , [41] . However, of these residues only Asn131, Phe382 and Asn391 are unique to LCAT, indicating that other residues in this region may simply play a structural role. The functional role of this region and how ApoA-I binding at this site might lead to LCAT activation remains to be determined. In summary, the crystal structures of LPLA2 and LCAT have revealed the unique architecture of a small family of lipid metabolizing enzymes that play important roles in human physiology and disease. Immediate goals are to determine a high-resolution structure of LCAT, to understand the molecular rules for substrate selectivity, and to better define the roles of LPAL2-Asp13 and LCAT-Cys31, which, along with the studies presented here, could be used to design improved therapeutics to treat FED, FLD and cholesterol-related disorders. These results also provide the foundation for the next generation of studies investigating how LCAT is activated by HDL particles and, in particular, by ApoA-I. Protein production Wild-type LPLA2 . The PCEP4 plasmid containing the human LPLA2 gene with codons optimized for expression in mammalian cell culture was obtained from Proteos (Kalamazoo, MI). The construct encodes full-length LPLA2 gene, including its signal sequence, followed by a 6xHis tag and tobacco etch virus (TEV) protease cleavage site, followed by sequence corresponding to mature LPLA2. For convenience, the construct was subcloned into the smaller pcDNA4 vector (pcDNA4-LPLA2). For expression of LPLA2, HEK293S GnTi − cells (ATCC) were grown in suspension in FreeStyle media (Gibco) supplemented with 0.5% fetal bovine serum. The cells were transiently transfected at a density of 1.5 × 10 6 ml −1 using a 1:2 molar ratio of pcDNA4-LPLA2:PEI and conditioned media was harvested 5 days later. SeMet-labelled LPLA2 . Because the yields of SeMet-labelled LPLA2 (SeMet-LPLA2) from transiently transfected HEK293S GnTi- cells was very low (150 μg l −1 ), a stable cell line for SeMet-LPLA2 expression was created. HEK293S GnTi − cells were grown as an adherent monolayer in DMEM high-glucose media, supplemented with 10% fetal bovine serum, 1 mM pyruvate, 2 mM L -glutamine, 100 U ml −1 penicillin and 100 μg ml −1 streptomycin. One day after transient transfection, media were exchanged and zeocin was added to 50 μg ml −1 final concentration. After cells were recovered, selection pressure was increased to 200 μg/ml zeocin in 50 μg/ml steps. At this step, protein yield for unlabelled LPLA2 was about 6 mg l −1 (38 × 150 mm 2 plates). Seven plates of stably transfected HEK293S GnTi − cells were then grown in the presence of 200 μg ml −1 zeocin to 90–95% confluence, then split into 38 plates without antibiotic and grown for an additional 3 days to 100% confluence. Subsequently, the cells were grown in complete medium supplemented with 30 mg l −1 SeMet and harvested after 3 days. LCAT . The human LCAT gene was optimized for expression in mammalian cell culture (Invitrogen) and then subcloned into the pcDNA4 vector. The LCAT FL construct was created by adding 6xHis to the C terminus using QuikChange. The ΔNΔC LCAT construct (LCAT 21–397 ) was created by deleting nucleotides encoding amino acids 1–20 and 398–416 of mature signal processed LCAT FL . LCAT FL and LCAT 21–397 were expressed by transient transfection of HEK293F cells (Invitrogen). Protein purification Media from cells expressing LPLA2 or LCAT was supplemented with HEPES pH 7.5 to a final concentration of 50 mM and then loaded on a 3-ml Ni-NTA-column. After washing with 100 ml buffer containing 20 mM HEPES pH 7.5, 300 mM NaCl and 10 mM imidazole pH 8, LPLA2 was eluted using the same buffer containing 200 mM imidazole pH 8. TEV (5% of total protein) and a 1:10 molar ratio of endoF1:LPLA2 were added to the eluate and the protein was dialysed overnight at 4 °C against 20 mM HEPES pH 7.5, 100 mM NaCl and 1 mM DTT. The protein was then passed through a second Ni-column to remove the cleaved His tag and undigested protein. The flow-through was further dialysed against 20 mM HEPES pH 7.5 and 150 mM NaCl and then concentrated to 13 mg ml −1 . Yields were about 2 mg l −1 of media for unlabelled LPLA2 using the transient expression method and about 1 mg l −1 of media for SeMet-LPLA2 produced in stably transfected cells. SeMet incorporation was confirmed using electrospray mass spectrometry with positive ion detection of the intact protein, wherein four separate peaks corresponding to 8, 7, 6 and 5 methionines of LPLA2 being substituted with SeMet were observed (mature LPLA2 has eight methionines). From the relative peak heights, the total incorporation was estimated to be 70–80%. LCAT FL and LCAT 21–397 was purified similarly to LPLA2, but the endoF1 and TEV digests were omitted as well as the second Ni-column purification step. Yields were 1.5–2 mg l −1 of media. Protein derivatization for crystallization For covalent modification with IDFP or MAFP, 50 μM fluorophosphonate inhibitor (Cayman chemical) was incubated with 0.4 mg ml −1 LPLA2 for 1 h at room temperature, and then LPLA2 was concentrated to 10–13 mg ml −1 . Crystallization LPLA2 and SeMet-LPLA2 were crystallized by vapour diffusion in hanging drops over reservoirs containing 100 mM HEPES pH 7.5, 3.5% PEG 8000, 28% MPD and 300 mM ammonium phosphate. If crystals did not appear after 5 days, they were streak seeded using smaller LPLA2 crystals obtained at higher MPD and PEG concentrations. P 1 LPLA2·IDFP and LPLA2·MAFP data sets were obtained by soaking LPLA2 crystals in harvesting solution containing 1 mM IDFP or MAFP for 2 days, and then freezing the crystals on nylon loops in liquid N 2 . The P 4 3 2 1 2 LPLA2·MAFP data set was obtained from a crystal grown using MAFP-modified LPLA2 and a condition from the Index HT screen (Hampton): 100 mM HEPES pH 7.5, 30% PEG MME 550, 50 mM MgCl 2 . Crystals of LPLA2-S165A were grown using a condition from the Classics Lite Suite (Qiagen): 100 mM Na cacodylate pH 6.5, 10% PEG 8000, 200 mM MgAc 2 and cryoprotected in solution containing 100 mM Na cacodylate pH 6.5, 50 mM Na citrate pH 4.5, 20 mM HEPES pH 7.5, 10% PEG 8000, 200 mM MgAc 2 and 30% ethylene glycol. Glycosylated LPLA2 produced in HEK293S GnTi − (without endoF1 treatment) was crystallized in 100 mM citric acid pH 3, 0.8 M ammonium sulfate in a condition derived from the JCSG+ screen (Qiagen). Cryoprotection was achieved by a solution containing 30% glycerol, 20 mM HEPES pH7.5, 150 mM NaCl, 100 mM citric acid pH 3 and 0.8 M ammonium sulfate. Crystals of fully glycosylated LPLA2 expressed in HEK293T cells (Proteos), purified as described for LCAT 21–397 , grew in 100 mM Na citrate pH 3.5–4, 20% PEG 3350 and 100 mM NaCl. Crystals were cryoprotected by soaking in solution containing 20% glycerol, 20 mM HEPES pH7.5, 150 mM NaCl, 100 mM Na citrate pH 4, 20% PEG 3350 and 100 mM NaCl. LCAT 21–397 was crystallized in 100 mM Na acetate pH 5.0, 13% isopropanol and 200 mM CaCl 2 . Cryoprotection was achieved by adding dry glucose to a final concentration of 30% (w/v) in mother liquor. Structure determination and refinement Data were collected at the Advanced Photon Source at Argonne National Laboratories on either the GM/CA or LS-CAT beam lines from crystals frozen in nylon cryoloops (Hampton). LPLA2, LPLA2-S165A and LPLA2·MAFP (HEK293S GnTI − without endoF1 treatment) data sets were collected at 0.97937 Å; LPLA2-IDFP and LPLA2-MAFP at 0.97857 Å; P 4 3 2 1 2 LPLA2-MAFP and LPLA2 (HEK293T) at 0.97933 Å; and LCAT 21–397 at 0.97857 Å. For experimental phase determination, the SeMet-LPLA2 data set was collected using a 10 μM mini-beam and vector data collection at GM/CA CAT. Data were integrated using XDS [42] and merged with SCALA in the CCP4 suite [43] . The selenium substructure, consisting of 32 Se sites (four LPLA2 molecules per asymmetric unit with eight methionines in each), was identified using ShelxD [44] and initial phases (figure of merit=0.35) were determined by single anomalous diffraction in AutoSol as implemented in the Phenix software package [45] . The initial atomic model was created with Phenix AutoBuild. All other data sets were scaled using the HKL2000 package [46] and merged with Aimless in the CCP4 suite. The preliminary SeMet-LPLA2 structure was used as a search model in molecular replacement using PHASER [47] to solve the remaining LPLA2 structures. Refinement was performed with alternating rounds of TLS and restrained refinement in REFMAC5 (ref. 48 ) and model building in Coot [49] . During refinement, local NCS restraints were applied when appropriate. MAFP density was not observed in the P 4 3 2 1 2 LPLA2·MAFP and LPLA2·MAFP (HEK293S GnTI − ) structures. Ramachandran statistics: 97.5% (favoured)/0% (outliers), 97.6/0.1%, 97.9/0%, 98/0%, 97.6/0%, 97.3/0.3% and 97.5/0% corresponding to the LPLA2, LPLA2·IDFP, LPLA2-S165A, P 4 3 2 1 2 LPLA2·MAFP, LPLA2·MAFP (HEK293S GnTI − ), LPLA2 (HEK293T) and P 1 LPLA2·MAFP structures, respectively. To determine the LCAT 21–397 structure, the LPLA2 model was truncated to the last common Cβ used as a search model in PHASER. An LPLA2-based homology model, built using the UCSF Chimera package [50] , was then superimposed onto the solution and used as the starting point for structure refinement. Fourfold NCS restraints were applied during refinement with restrained and jelly body refinement in REFMAC. Despite observed density for the C-terminal His tag, it was left unmodelled. Ramachandran statistics: 94.9% (favoured)/0.3% (outliers). All models were validated for stereochemical correctness using MolProbity [51] . pNPB hydrolysis pNPB (Sigma) was diluted to 10 mM using the reaction buffer (20 mM HEPES pH 7.5, 150 mM NaCl) containing 10% dimethylsulphoxide, and the reaction was started by addition of 40 μl 0.1 μM LPLA2 to 10 μl of pNPB. Release of the p -nitrophenoxide was monitored by increased absorbance at 400 nm on a Spectramax plate reader. Data from at least three independent experiments were analysed with paired t-test in GraphPad Prism. Differential scanning fluorimetry LPLA2 or LCAT variant (0.1 mg ml −1 ) was mixed with 0.1 mM 1-anilinonaphthalene- 8-sulfonic acid in the absence and presence of 100 μM IDFP or MAFP in 20 mM HEPES pH 7.5 and 150 mM NaCl. Samples were heated from 25 to 90 °C at 1 °C min −1 in a ThermoFluor Analyzer (Johnson & Johnson). Plate fluorescence was measured in 1°C intervals after cooling to 25 °C using a 475–525 nm emission filter. T m values were calculated as the inflection point of the melting curve using the instrument software. Liposome-based activity assays The transacylase activity assay of LPLA2 was performed using a reaction mixture containing 48 mM Na citrate pH 4.5, 10 μg ml −1 bovine serum albumin and liposomes (127 μM phospholipid) and LPLA2 in 500 μl of total volume. Liposomes consisting of DOPC-sulfatide-NAS (3:0.3:1, molar ratio) were prepared as previously described [52] . The LPLA2 concentration was 30 ng ml −1 . The reaction was initiated by the addition of the enzyme. The reaction mixture was incubated for 30 min at 37 °C and terminated by adding 3 ml of chloroform-methanol (2:1) plus 0.3 ml of 0.9% (w/v) NaCl. The mixture was centrifuged for 5 min at room temperature. The resulting lower organic layer was transferred into another glass tube and dried under a stream of N 2 gas. The dried lipid was dissolved in 40 μl of chloroform-methanol (2:1) and applied on an HPTLC plate and developed in a solvent system consisting of chloroform-acetic acid (90:10, v/v). The plate was dried and soaked in 8% (w/v) CuSO 4 ·5H 2 O, 6.8% (v/v) H 3 PO 4 , 32% (v/v) methanol. The uniformly wet plate was briefly dried by a hair dryer and charred for 15 min in a 150 °C oven. The plate was scanned and the content of the product (1-O-acyl-NAS) was estimated by NIH-ImageJ 1.37v. For the phospholipid esterase activity assay, liposomes consisting of DOPC-sulfatide (10:1, molar ratio) without NAS were used. Although the formation of lyso-PC could be detected with a low concentration of LPLA2 (30 ng ml −1 ), a concentration of 10 μg ml −1 was used to ensure that residual activity of LPLA2 variants could be detected. Liposome co-sedimentation Liposomes consisting of DOPC or DODPC-sulfatide (10:1, molar ratio, 127 μM total) were incubated with 7.2 μg of recombinant mouse LPLA2 or MAFP-modified LPLA2 in 500 μl of 48 mM Na citrate pH 4.5 for 30 min on ice. The reaction mixture was then centrifuged for 1 h at 150,000 g at 4 °C. The resulting precipitate was briefly rinsed with cold 50 mM Na citrate pH 4.5 and dissolved with 40 μl of SDS-polyacrylamide gel electrophoresis sample buffer. The sample was separated by using 12% SDS-polyacrylamide gel electrophoresis. After electrophoresis, LPLA2 was detected with Coomassie brilliant blue. Band quantification was performed with ImageJ software. Figures Molecular graphics and visualization were performed using the PyMOL Molecular Graphics System (Schrödinger, LLC). Electrostatic calculations were performed using the PDB2PQR server [53] and the APBS plugin [54] for PyMOL. Accession codes . Atomic coordinates and structure factors are deposited in the Protein Data Bank ( http://pdb.rcsb.org ) as entries 4X90 , 4X91 , 4X92 , 4X93 , 4X94 , 4X95 , 4X96 , 4X97 , corresponding to the LPLA2, LPLA2·IDFP, LPLA2-S165A, P43212 LPLA2·MAFP, LPLA2·MAFP (HEK293S GnTI-), LPLA2 (HEK293T), LCAT21-397, and P1 LPLA2·MAFP structures, respectively. How to cite this article: Glukhova, A. et al . Structure and function of lysosomal phospholipase A2 and lecithin:cholesterol acyltransferase. Nat. Commun. 6:6250 doi: 10.1038/ncomms7250 (2015).